Specific inhibition of bacterial RNase T2 by helix 41 of 16S ribosomal RNA Ribonuclease (RNase) T2 is involved in scavenging exogenous RNAs in the periplasmic space of bacteria. In Escherichia coli , although the 30S ribosomal subunit has long been known as a specific inhibitor of RNase T2 (designated as RNase I in E. coli ), both the biochemical mechanisms and physiological roles of this interaction remain to be elucidated. Here we show, by creating hybrid ribosomes and mutational studies, that helix 41 (h41) of the E. coli 16S ribosomal RNA has a crucial role in the specific inhibition of RNase I. Notably, h41-mutant strains exhibit a lower survival rate at stationary phase and severe cell lysis when the post-segregation killing protein SrnB is expressed. These phenotypic defects accompany significant RNA degradation caused by RNase I. Thus, h41 in 16S rRNA provides a physiological benefit for the host cells in coping with the potential cytotoxicity of RNase T2. Ribonuclease (RNase) T2 was first discovered in Aspergillus oryzae (Taka-diastase) [1] , which is a single-strand-specific, transferase-type endonuclease that cleaves RNA at all dinucleotide bonds, leaving a 5′-hydroxyl and 2′-,3′-cyclic monophosphate [2] . RNase T2 genes are found in the genomes of bacteria, fungi, protozoans, animals, plants and viruses and this group represents one of the most widely distributed RNase families [2] . In these organisms, RNase T2 is generally localized in an extracellular space (that is, periplasmic space of Gram-negative bacteria) or membrane-bound compartments such as lysosome or vacuole [2] . An important role of RNase T2 is scavenging extracellular RNAs to supply nutrients for the cell. For example, when tomato cells are starved for phosphate, cells secrete RNase LE to digest extracellular RNAs and incorporate the digests as a phosphate source [3] , [4] . A similar phenomenon is observed in the human intestinal pathogen Entamoeba histolytica [5] . While RNase T2 may nutritionally benefit the cell, this enzyme also has potential cytotoxicity. For example, when Saccharomyces cerevisiae cells are subjected to oxidative stress, Rny1 leaks from the vacuole to the cytoplasm and digests cellular transfer RNAs and ribosomal RNAs, leading to cell death [6] , [7] . In swine fever virus or bovine viral diarrhoea virus, the envelope protein E rns contains an RNase T2 domain that may perturb the host's immune cells [8] , [9] . Plants even exploit the cytotoxicity of RNase T2 to prevent self-fertilization [10] . In the gametophytic self-incompatibility system of Solanaceae, Rosaceae and Plantaginaceae, elongation of the incompatible (self) pollen tube through the styles is strongly inhibited by S-RNase (the female component) that enters, from the extracellular matrix of styles, to the pollen tube and thereby degrades rRNAs. When compatible (non-self) pollen elongates, however, S-RNase activity is specifically prevented by the male component, which is now putatively identified as a ubiquitin ligase [10] . In Escherichia coli , the homologue of RNase T2 is traditionally called RNase I, which is present in the periplasmic space as a 27-kDa monomer [11] , [12] , [13] . RNase I is unique in that it does not require Mg 2+ for activity; in the presence of EDTA, ∼ 99% of the total RNase activity is due to RNase I (refs 13 , 14 ). Moreover, despite the periplasmic localization of RNase I, the ribosomal 30S subunit in the cytosol has been shown in vitro to possess binding/inhibitory activity for RNase I (refs 15 , 16 , 17 , 18 ), whiereas the 50S particle does not [18] unless specially treated [19] . Detailed biochemical studies, however, revealed that neither naked 16S rRNA nor total ribosomal proteins (TP30) independently inhibited RNase I (ref. 18 ). Thus, the 30S subunit, as a ribonucleoprotein particle, probably specifically binds to/inhibits RNase I. In terms of cellular physiology, the existence of RNase I-inhibitors has been predicted. For example, when E. coli cells are treated with Hg 2+ , a putative RNase I-inhibitor is inactivated, and RNase I breaks down significant quantities of rRNAs and tRNAs [20] , which is consistent with the report stating that expression of recombinant RNase I in E. coli does not show the expected activity as compared with that of other recombinant RNases [21] . However, whether the Hg 2+ -sensitive RNase I-inhibitor is related to the 30S subunit or two independent RNase I-inhibitors exist in E. coli remains unknown. In this paper, we first created hybrid 30S subunits in which only the 16S rRNAs were exchanged for homologues of distantly related bacteria, and showed that the 16S rRNA sequence is critical for RNase I-inhibition. Domain replacement, helix swapping and mutational studies at the single-nucleotide level showed that helix 41 (h41) in the 16S rRNA is the specific determinant of inhibition. An h41 mutant of E. coli showed a clearly defective phenotype, demonstrating the biochemical and physiological significance of the specific interaction between h41 and RNase I. RNA degradation in E. coli carrying foreign 16S rRNA First, to introduce a large perturbation in the 30S ribosomal subunit, we focused on the 16S rRNA, the major constituent of the 30S subunit, which was replaced with those from non- E. coli bacteria, generating a hybrid ribosome. To fully replace E. coli 16S rRNA, we used a mutant E. coli strain KT101 in which all chromosomal rrn operons were deleted and compensated by a rescue plasmid pRB101 (refs 22 , 23 ). As donors of 16S rRNA genes, we selected two bacteria, Serratia ficaria (denoted as Sfi) and Ralstonia pickettii (Rpi), as well as E. coli (Eco) as the positive control ( Fig. 1a ). Using the plasmid replacement technique [22] , we obtained the E. coli strains KT103/Sfi, KT103/Rpi, KT103/Eco that contained the 16S rRNA genes from Sfi, Rpi and Eco, respectively ( Fig. 1a ). KT103/Sfi displayed only a moderate growth defect (doubling time: 40.7±1.9 min) as compared with that of KT103/Eco (34.5±0.2 min). In contrast, KT103/Rpi exhibited a more severe growth defect (59.5±8.3 min), resulting in small colonies on a Luria–Bertani (LB) agar plate containing sucrose ( Fig. 1a ). 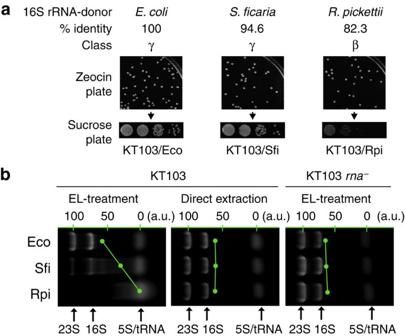Figure 1: RNA degradation inE. colicarrying foreign 16S rRNA. (a) Functional complementation ofE. coliKT101 cells. pRB103 constructs with non-E. coli16S rRNA genes were used to transformE. coliKT101. To completely exclude the rescue plasmid pRB101, transformants selected on Zeocin plates were serially diluted (to 103–106) and spotted onto sucrose plates. '% identity' denotes the nucleotide identities betweenE. coliand non-E. coli16S rRNA sequences; 'class' denotes phylogenetic classes within the phylum Proteobacteria. (b) Electrophoresis patterns of total RNA extracted from KT103 cells. Total RNA was extracted and analysed by denaturing agarose gel electrophoresis. A green dot in each lane represents the centre of the RNA mass (xcentre), which is used as the degradation index (Methods). Locations of bands corresponding to 23S rRNA and 5S rRNA/tRNAs were defined as 100 and 0 (arbitrary units, a.u.), respectively, and are shown at the top of the gel. Figure 1: RNA degradation in E. coli carrying foreign 16S rRNA. ( a ) Functional complementation of E. coli KT101 cells. pRB103 constructs with non- E. coli 16S rRNA genes were used to transform E. coli KT101. To completely exclude the rescue plasmid pRB101, transformants selected on Zeocin plates were serially diluted (to 10 3 –10 6 ) and spotted onto sucrose plates. '% identity' denotes the nucleotide identities between E. coli and non- E. coli 16S rRNA sequences; 'class' denotes phylogenetic classes within the phylum Proteobacteria. ( b ) Electrophoresis patterns of total RNA extracted from KT103 cells. Total RNA was extracted and analysed by denaturing agarose gel electrophoresis. A green dot in each lane represents the centre of the RNA mass ( x centre ), which is used as the degradation index (Methods). Locations of bands corresponding to 23S rRNA and 5S rRNA/tRNAs were defined as 100 and 0 (arbitrary units, a.u. ), respectively, and are shown at the top of the gel. Full size image To investigate how these replacements affected the RNase I-inhibitor activity of the 30S subunit, we performed an RNA extraction assay to analyse the degradation of total cellular RNAs (mainly rRNAs and tRNAs). In this assay, two different RNA extraction methods were used, the EDTA–lysozyme (EL) method and the direct extraction method, and the resulting electrophoretic patterns of RNA were compared. Although roughly the same yield of total cellular RNAs was obtained regardless of the extraction method (data not shown), we noticed that their electrophoretic patterns were quite different ( Fig. 1b; Supplementary Fig. S1 ). To quantify the degree of RNA degradation, the centre of the RNA mass ( x centre , defined in Methods) was calculated for each lane and marked by green dots on the gel. With the EL method, three RNA bands that corresponded to the 23S rRNA, 16S rRNA and 5S rRNA/tRNAs, respectively, were detected for KT103/Eco ( x centre =56.3). In contrast, moderate ( x centre =30.5) and heavy ( x centre =1.0) degradation was observed for KT103/Sfi and KT103/Rpi, respectively ( Fig. 1b ). This difference was not observed for any of the mutants with the direct extraction method ( Fig. 1b ). Notably, when KT103 rna − , whose RNase I gene ( rna ) had been disrupted [22] , was used as a host strain, no degradation occurred even with the EL method ( Fig. 1b ), confirming that the degradation was due solely to RNase I. h41 is responsible for RNase I-inhibition To specify the RNA domain responsible for RNase I-inhibition, we next created chimeric 16S rRNAs between Eco and either Sfi or Rpi. We targeted the 3′-major domain (U921-A1396, 476 bp) ( Fig. 2a ) and substituted it with the corresponding region of Sfi 16S rRNA (7.1% difference). RNA extraction analysis of KT103 containing this construct (KT103/Eco ∷ Sfi) by the EL method showed a moderate degree of degradation ( x centre =32.2) ( Fig. 2b ), suggesting that the 3′-major domain is responsible for inhibition. We also created another chimeric 16S rRNA gene containing the 3′-major domain of Rpi 16S rRNA, whose sequence was more radically (20.2%) different (Eco ∷ Rpi). In this case, a more severe degradation ( x centre =0.0) was observed ( Fig. 2b ). Such degradation was not detected for any variant using the direct extraction method, or even the EL-treatment method if KT103 rna − cells were used ( Fig. 2b ). The importance of the 3′-major domain was further supported by using Rpi 16S rRNA, the 3′-major domain of which had been substituted with that of Eco (Rpi ∷ Eco); RNA instability was significantly ameliorated ( x centre =43.4) ( Fig. 2b ). 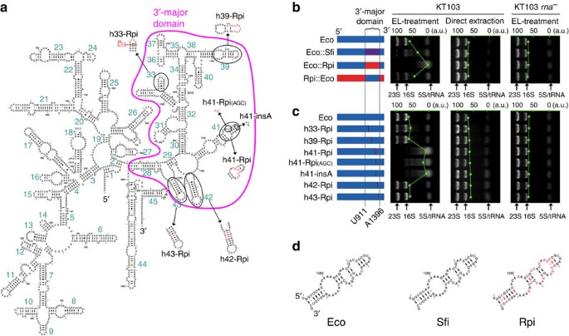Figure 2: h41 is responsible for RNase I-inhibition. (a) Secondary structure ofE. coli16S rRNAs. The secondary structure map was obtained from the Comparative RNA website and project (http://www.rna.ccbb.utexas.edu/). The 3′-major domain (U921-A1396, 476 bp) is encircled in pink. All RNA helices (h1–h45) are numbered and helices that were altered to Rpi sequences are circled with Rpi sequences. (b) Electrophoresis patterns of total RNA from KT103 cells harbouring 16S rRNA genes with various substituted 3′-major domains. (c) Narrowing down the inhibitory region within the 3′-major domain of Eco 16S rRNA by replacing RNA helices with the corresponding region of Rpi sequences. (d) Secondary structures of h41 of Eco, Sfi and Rpi. As compared with the Eco sequence, bases that are different in the Sfi and Rpi sequences are coloured purple and red, respectively. (b,c) A green dot in each lane represents the centre of the RNA mass (xcentre), which is used as the degradation index (seeMethods). Locations of bands corresponding to 23S rRNA and 5S rRNA/tRNAs were defined as 100 and 0 (arbitrary units, a.u.), respectively, and are shown at the top of the gel. Figure 2: h41 is responsible for RNase I-inhibition. ( a ) Secondary structure of E. coli 16S rRNAs. The secondary structure map was obtained from the Comparative RNA website and project ( http://www.rna.ccbb.utexas.edu/ ). The 3′-major domain (U921-A1396, 476 bp) is encircled in pink. All RNA helices (h1–h45) are numbered and helices that were altered to Rpi sequences are circled with Rpi sequences. ( b ) Electrophoresis patterns of total RNA from KT103 cells harbouring 16S rRNA genes with various substituted 3′-major domains. ( c ) Narrowing down the inhibitory region within the 3′-major domain of Eco 16S rRNA by replacing RNA helices with the corresponding region of Rpi sequences. ( d ) Secondary structures of h41 of Eco, Sfi and Rpi. As compared with the Eco sequence, bases that are different in the Sfi and Rpi sequences are coloured purple and red, respectively. ( b , c ) A green dot in each lane represents the centre of the RNA mass ( x centre ), which is used as the degradation index (see Methods ). Locations of bands corresponding to 23S rRNA and 5S rRNA/tRNAs were defined as 100 and 0 (arbitrary units, a.u. ), respectively, and are shown at the top of the gel. Full size image To further identify the core inhibitor region within the 3′-major domain, we systematically swapped RNA helices that were variable between Eco and Rpi 16S rRNAs: helices (h) 33, 39, 41, 42 and 43 ( Fig. 2c ). Using an RNA extraction assay, we found that significant RNA degradation ( x centre =7.6) occurred only when h41 was replaced with the Rpi sequence (h41-Rpi) ( Fig. 2c,d ). By mutating h41, we found that one variant, h41-Rpi (AGC) ( Fig. 2a ), in which only three bases of the Eco were altered to those of the Rpi sequence (C1262A, C1263G and U1264C), showed severe RNA degradation ( x centre =16.8) ( Fig. 2c ). Moreover, a mutant h41-insA ( Fig. 2a ), in which one adenine base was inserted in the loop of h41 (between C1267 and G1268), also caused severe degradation ( x centre =7.1) ( Fig. 2c ). Notably, these KT103 mutants showed healthy growth in the exponential phase (doubling times: 37.0±0.4 min for h41-Rpi (AGC) and 34.8±0.4 min for h41-insA), suggesting that the loss of RNase I-inhibitor activity was not due to loss of functionality of the ribosome. Again, no degradation was observed for any of these variants with the direct extraction method or the EL method of KT103 rna − cells ( Fig. 2b,c ). These data strongly suggest that the identity of the h41 sequence was critical for the RNase I-inhibition. RNase I is inhibited through specific interactions with h41 We next performed in vitro studies using recombinant RNase I and purified 30S subunits. 30S subunits (30S/Eco, Sfi and Rpi) were isolated from KT103 rna − cells that contained the 16S rRNAs of Eco, Sfi and Rpi, respectively. We also prepared the 30S subunit (30S/h41-Rpi) from KT103 rna − with a chimeric 16S rRNA (h41-Rpi). Recombinant RNase I was then mixed with these subunits, and the remaining RNase activities were determined using the RNase Alert Lab Test Kit. In this experiment, a fluorescent and quencher-labelled RNA was used as an external substrate, and RNase activity was measured by detecting liberated fluorescence. Compared with the 50S subunit (negative control; no RNase I-inhibitor activity [18] ), we found that 30S/Eco strongly inhibited RNase activity, whereas 30S/Sfi displayed moderate inhibitory activity and that of 30S/Rpi and 30S/h41-Rpi was weak ( Fig. 3a,b ). Naked 16S rRNAs extracted from 30S/Eco or 30S/Rpi did not inhibit RNase I activity ( Supplementary Fig. S2 ). When bovine pancreatic RNase A was used instead of RNase I, no difference in the inhibitory effects of the four 30S subunits was observed ( Fig. 3c ), indicating that h41-mediated inhibition is specific to RNase I. 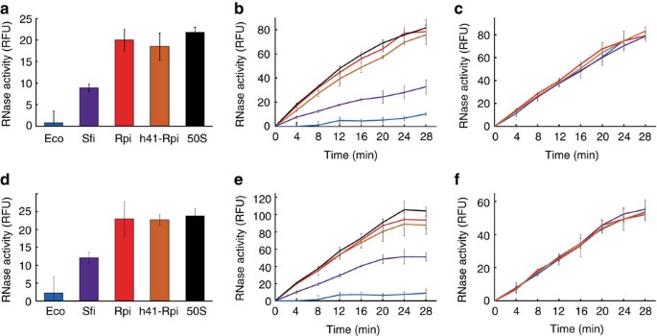Figure 3: RNase I is inhibited through specific interactions with h41. (a–c)In vitroinhibition assay. Hybrid 30S subunits with various 16S rRNAs were purified from KT103rna−cells and mixed with recombinant RNase I; the RNase activity (a) after 6-min incubation and (b) the time course was determined. (c) Control experiment using RNase A. 30S subunits were mixed with 0.25 pg of recombinant RNase A. (d–f)In vitrobinding assay. Hybrid 30S subunits were mixed with recombinant RNase I and passed through an ultrafiltration membrane (100 kDa cutoff). The flow-through fraction (presumed to contain free RNase I) was used to determine RNase activity (d) after 6-min incubation and (e) the time course was determined. (f) Control experiment using RNase A. 30S subunits were mixed with 0.25 pg of recombinant RNase A. (a–f) RNase activity was determined using the RNase Alert Lab Test Kit. Fluorescence (RFU) was monitored on a SPECTRAmax GEMINI XS spectrofluorometer at excitation/emission wavelengths of 490 nm and 520 nm, respectively. (b,c,e,f) Lines: blue, Eco; purple, Sfi; red, Rpi; orange, h41-Rpi; black, 50S (control). Error bars represent the standard deviation of three replicate reactions. Figure 3: RNase I is inhibited through specific interactions with h41. ( a–c ) In vitro inhibition assay. Hybrid 30S subunits with various 16S rRNAs were purified from KT103 rna − cells and mixed with recombinant RNase I; the RNase activity ( a ) after 6-min incubation and ( b ) the time course was determined. ( c ) Control experiment using RNase A. 30S subunits were mixed with 0.25 pg of recombinant RNase A. ( d–f ) In vitro binding assay. Hybrid 30S subunits were mixed with recombinant RNase I and passed through an ultrafiltration membrane (100 kDa cutoff). The flow-through fraction (presumed to contain free RNase I) was used to determine RNase activity ( d ) after 6-min incubation and ( e ) the time course was determined. ( f ) Control experiment using RNase A. 30S subunits were mixed with 0.25 pg of recombinant RNase A. ( a – f ) RNase activity was determined using the RNase Alert Lab Test Kit. Fluorescence (RFU) was monitored on a SPECTRAmax GEMINI XS spectrofluorometer at excitation/emission wavelengths of 490 nm and 520 nm, respectively. ( b , c , e , f ) Lines: blue, Eco; purple, Sfi; red, Rpi; orange, h41-Rpi; black, 50S (control). Error bars represent the standard deviation of three replicate reactions. Full size image To confirm that RNase I binds to the 30S subunit on inhibition, we performed an in vitro binding assay. RNase I and the 30S subunit were mixed and then subjected to ultrafiltration (100 kDa, cutoff). The activity of free (nonbinding) RNase I (67 kDa as a fusion with maltose-binding protein) was detected from the flow-through fraction ( Fig. 3d,e ). Compared with the control using the 50S subunit, which does not interact with RNase I (ref. 18 ), we found that 30S/Eco interacted significantly with RNase I, but that 30S/Rpi and 30S/h41-Rpi did not ( Fig. 3d,e ). When similar experiments were performed with RNase A, no such difference among the four 30S subunits was observed ( Fig. 3f ). Thus, h41 was suggested to interact specifically with RNase I on inhibition. Phenotypes of E. coli carrying 16S rRNA with altered h41 We investigated the physiological significance of the interaction between h41 and RNase I on growth phenotype. KT103/Eco and KT103/h41-Rpi showed no significant differences in exponential growth ( Fig. 4a ). However, after prolonged cultivation (24 h), the viability of KT103/h41-Rpi decreased significantly (41.7% reduction as compared with KT103/Eco) ( Fig. 4a ), which accompanied RNA degradation ( x centre =15.1) ( Fig. 4b ). Such phenotypes were not observed in KT103 rna − cells ( Fig. 4a,b ). A possible explanation for this phenomenon is that increased membrane permeability, which is known to occur in stationary phase [11] , [24] , induced the entry of periplasmic RNase I into the cytoplasm, resulting in RNA instability and growth defect in the absence of RNase I-inhibitor (h41). 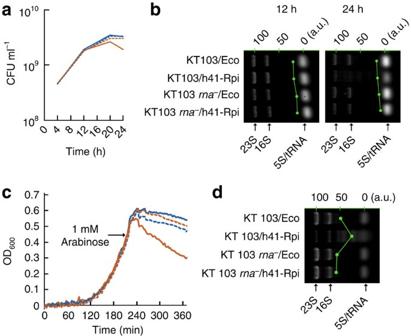Figure 4: Phenotypes ofE. colicarrying 16S rRNA with altered h41. (a) Growth curves. KT103 or KT103rna−cells with or without the h41 mutation were cultured for 24 h and the numbers of colony forming units (CFU) ml−1were plotted. (b) RNA degradation observed for h41 mutant cells in stationary phase. Cells were collected after 12 and 24 h (stationary phase) and the total RNA was prepared by direct extraction, followed by denaturing agarose gel electrophoresis. (c) Growth curves of KT103 cells expressing the SrnB toxin. Growth was monitored in real-time using an ODMonitor AS. When cell density reached OD600=0.45, arabinose was added to the medium to induce the expression of SrnB. (d) RNA degradation in KT103 with mutant h41 after induction of SrnB. Cells were collected 15 min after induction. RNA was prepared by the direct extraction method and electrophoresed in a denaturing agarose gel. (a,c) Lines: KT103/Eco (blue solid), KT103/h41-Rpi (orange solid), KT103rna−/Eco (blue broken), KT103rna−/h41-Rpi (orange broken). (b,d) A green dot in each lane represents the centre of the RNA mass (xcentre), which is used as the degradation index (Methods). Locations of bands corresponding to 23S rRNA and 5S rRNA/tRNAs were defined as 100 and 0 (arbitrary units, a.u.), respectively, and are shown at the top of the gel. Figure 4: Phenotypes of E. coli carrying 16S rRNA with altered h41. ( a ) Growth curves. KT103 or KT103 rna − cells with or without the h41 mutation were cultured for 24 h and the numbers of colony forming units (CFU) ml −1 were plotted. ( b ) RNA degradation observed for h41 mutant cells in stationary phase. Cells were collected after 12 and 24 h (stationary phase) and the total RNA was prepared by direct extraction, followed by denaturing agarose gel electrophoresis. ( c ) Growth curves of KT103 cells expressing the SrnB toxin. Growth was monitored in real-time using an ODMonitor AS. When cell density reached OD 600 =0.45, arabinose was added to the medium to induce the expression of SrnB. ( d ) RNA degradation in KT103 with mutant h41 after induction of SrnB. Cells were collected 15 min after induction. RNA was prepared by the direct extraction method and electrophoresed in a denaturing agarose gel. ( a , c ) Lines: KT103/Eco (blue solid), KT103/h41-Rpi (orange solid), KT103 rna − /Eco (blue broken), KT103 rna − /h41-Rpi (orange broken). ( b , d ) A green dot in each lane represents the centre of the RNA mass ( x centre ), which is used as the degradation index (Methods). Locations of bands corresponding to 23S rRNA and 5S rRNA/tRNAs were defined as 100 and 0 (arbitrary units, a.u. ), respectively, and are shown at the top of the gel. Full size image To directly demonstrate that membrane-damage decreases the probability of bacterial survival in the presence of RNase I and absence of h41, we expressed SrnB, an F-factor-derived toxin that depolarizes the inner membrane [25] , [26] , during mid-log phase in KT103 cells. Only KT103/h41-Rpi showed severe cell lysis ( Fig. 4c ), which accompanied RNA degradation ( x centre =26.1) ( Fig. 4d ), strongly suggesting a model in which h41 in the 30S subunit protects cellular RNA (rRNA and tRNA) from RNase I entry when the inner membrane is damaged (that is, aged, depolarized or injured) ( Fig. 5 ). 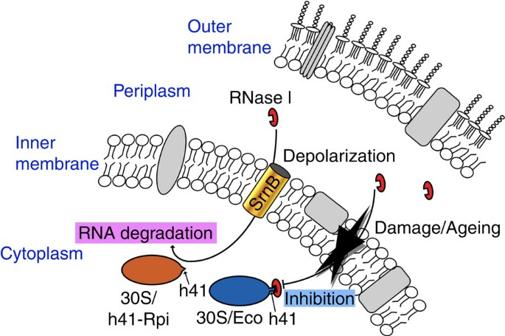Figure 5: Model of the functional interaction between RNase I and h41. RNase I is usually localized in the periplasmic space ofE. coli(∼220 molecules per single KT103 cell, calculated from the result inSupplementary Fig. S2). RNase I enters the cytoplasm when the inner membrane is aged, injured or depolarized. After entry to the cytoplasm, the activity of RNase I is inhibited by the ribosomal 30S subunit (∼21,700 particles per single KT103 cell, as calculated from OD260value) through specific binding. In this interaction, the identity of the h41 sequence in the 16S rRNA is responsible for both binding and inhibition. When h41 is mutated, the 30S subunit is no longer able to interact with RNase I, which then degrades cellular RNAs and perturbs the growth of the cell. Figure 5: Model of the functional interaction between RNase I and h41. RNase I is usually localized in the periplasmic space of E. coli ( ∼ 220 molecules per single KT103 cell, calculated from the result in Supplementary Fig. S2 ). RNase I enters the cytoplasm when the inner membrane is aged, injured or depolarized. After entry to the cytoplasm, the activity of RNase I is inhibited by the ribosomal 30S subunit ( ∼ 21,700 particles per single KT103 cell, as calculated from OD 260 value) through specific binding. In this interaction, the identity of the h41 sequence in the 16S rRNA is responsible for both binding and inhibition. When h41 is mutated, the 30S subunit is no longer able to interact with RNase I, which then degrades cellular RNAs and perturbs the growth of the cell. Full size image The primary function of 16S rRNA is to form the scaffold of the 30S ribosomal subunit, which is necessary for translating mRNA-encoded genetic information into proteins [27] , [28] . We here unveiled another function of 16S rRNA: an RNase inhibitor. To our knowledge, this is the first report showing a non-translational role of 16S rRNA. For several decades, biochemists have noticed that the 30S subunit binds to and inhibits RNase I (refs 15 , 16 , 17 , 18 , 24 ). Ribosomes are usually prepared from E. coli cells by disrupting by alumina-grinding or using a French press [29] . On disruption, RNase I in the periplasmic space mixes with the cytosol and inevitably attaches to 30S or 70S (30S+50S) particles in an inactive (latent) form, which can be reactivated to break down a significant amount of rRNAs, depending on Mg 2+ concentration [15] , [16] , [17] , [18] , [24] . Because of this phenomenon, RNase I was formerly called 'latent RNase' [15] or 'ribosomal RNase' [30] . However, the detailed mechanisms of the interaction between ribosomes and RNase I and its physiological meaning remained unclear for decades. We used the genetic system of E. coli KT101, which has an rna + genotype [22] , [23] , to show the involvement of 16S rRNA in the RNase I-inhibitory activity of the 30S subunit. In the replacement experiment ( Fig. 1a ), discovering that the hybrid ribosome containing 16S rRNA/Rpi can function in E. coli was unexpected, as 16S rRNA/Rpi has only an 80.5% sequence similarity to 16S rRNA/Eco (Squires' group has reported that the Proteus vulgaris rrn operon, which shows 93% similarity to that of Eco, can function in E. coli [31] ), strongly suggesting the architectural robustness of the ribosome (details will be published elsewhere). By using the EL method (and the direct extraction method as a control) in an RNA extraction assay, we found that the hybrid 30S subunit (30S/Rpi) had lost RNase I-inhibitor activity ( Fig. 1b ). The merit of using the EL method in the RNA extraction assay is to allow quantitation of net RNase I activity in a biologically significant stoichiometry, by simply mixing periplasmic RNase I and cytoplasmic RNAs (mainly rRNAs and tRNAs) for a relatively short time ( Supplementary Fig. S1 ). Although our method inevitably used 16S rRNA that was embedded in the 30S subunit both as a substrate and a possible inhibitor of RNase I, we also detected degradation of 23S rRNA or 5S/tRNAs as exterior substrates. Thus, loss of the RNase I-inhibitory activity of the 30S subunit was estimated as the decrease in the degradation index ( x centre , which is defined in the Methods) ( Figs 1 and 2 ). Results obtained by this analysis were concordant with the biochemical investigations, in which a fluorescent and quencher-labelled nonnatural RNA was used as an external substrate ( Fig. 3 ). By domain replacement and helix-swapping studies, followed by an RNA extraction assay, we identified h41 in 16S rRNA as the element responsible for RNase I-inhibitory activity ( Fig. 2 ). Much evidence indicates that h41 is directly involved in controlling RNase I activity ( Fig. 5 ). In the tertiary structure of the 30S ribosomal subunit, h41 locates at the top of the structure (the head) and protrudes to the exterior of the subunit [27] , [28] , potentially providing a direct binding site for RNase I. This direct interaction model is also supported by the fact that RNase I-inhibitory activity was significantly decreased by inserting even a single nucleotide to the tip of the hairpin, where no interactions are seen with other parts of 16S rRNA or ribosomal proteins [27] , [28] ( Fig. 2a,c ). Also, 30S/h41-Rpi is suggested to have lost both its RNase I-inhibitory activity and RNase I binding simultaneously ( Fig. 3 ). Moreover, we confirmed that loss of RNase I-inhibitory activity in the h41 mutant was not due to side effects of inefficient subunit assembly or the perturbation of certain ribosomal proteins, because the assembly ratios [22] , [32] and proteomic patterns of the 30S subunit (as observed by highly sensitive RFHR method of two-dimensional polyacrylamide gel electrophoresis) of 30S/Eco and 30S/h41-Rpi are virtually indistinguishable (K.K. and K.M., unpublished data). However, as reported previously [18] , we also confirmed that naked 16S rRNAs extracted from 30S/Eco or 30S/Rpi no longer inhibited RNase I activity ( Supplementary Fig. S2 ), seemingly conflicting with the direct interaction model ( Fig. 5 ). This fact suggests that the overall structure of the 30S particle acts as a scaffold for h41-mediated inhibition, or that h41-mediated RNase I-inhibition is assisted by the ribosomal proteins. Another possibility that cannot be completely excluded is that a ribosomal protein, which is either directly or indirectly affected by h41, is responsible for the inhibition. We experimentally clarified the physiological significance of the h41–RNase I interaction ( Fig. 4 ). Specifically, cells with altered h41 (KT103/h41-Rpi) showed RNA degradation and reduction of survival in the stationary phase (after 24 h cultivation) ( Fig. 4a,b ). We speculated that changes in KT103/h41-Rpi cell membrane permeability, which are known to occur on entry into stationary phase [11] , [24] , induced the entry of RNase I into the cytoplasm and resulted in RNA instability and a defect in growth. This was confirmed by a further experiment using SrnB, an F-factor-derived toxin that depolarizes the inner membrane and is known to induce entry of RNase I into the cytoplasm [25] , [26] ( Fig. 4c,d ). We observed clear phenotypic defects (that is, RNA degradation and cell lysis), suggesting that the RNase I-inhibitory activity in E. coli is mainly due to h41 within 30S subunit, and that the Hg 2+ -sensitive inhibitor [20] has a lesser physiological role. From these results, we propose a model in which h41, with the help of ribosomal proteins, protects cellular RNAs (rRNAs and tRNAs) from RNase I-attack when the inner membrane is damaged (that is, aged, depolarised or injured) ( Fig. 5 ). An example of a biological process in which RNA controls the activity of proteinaceous RNase is the ToxN–toxIN system in Erwinia carotovora [33] . Our findings should shed light on the origin and diversity of RNA-based RNase-inhibitors. Other than the functional implications, the 16S rRNA seems to be an ideal molecule to be used as an RNase inhibitor in terms of stoichiometry. We estimated that more than 20,000 particles of the 30S subunit exist in KT103 cells (as calculated from the amount of 16S rRNA; data not shown). However, only ∼ 200 molecules of RNase I are present in the periplasmic space of the same strain (as calculated by enzymatic activity; Supplementary Fig. S3 ). These values are roughly concordant with a previous study [16] . This is analogous to the eukaryotic cell that accumulates a significant amount of RNase A inhibitor, a protein with a molecular weight of ∼ 49 kDa that comprises ∼ 0.1% of total cellular protein mass [34] . Thus, this may represent a common strategy to protect cellular RNAs from highly active extracellular RNases by maintaining a sufficient quantity of inhibitors in the cytosol. According to the Pfam ( http://pfam.janelia.org/ ) [35] , RNase T2 family enzymes (PF00445) are distributed in many bacterial phyla (acidobacteria, actinobacteria, cyanobacteria and proteobacteria), fungi, protozoans, animals (including humans), plants and viruses [2] , but not in archaea. This is in contrast to the narrower distribution of other transferase-type RNases such as RNase A (animal-specific) and RNase T1 (mainly found in fungi) [2] . Thus, the inhibitory activity of RNase T2 can be reasonably assumed to be carried by another ancient molecule, the 16S rRNA. The secondary structure of h41 in the 16S rRNA is highly conserved among bacteria (see the Comparative RNA project; http://www.rna.ccbb.utexas.edu/ ) [36] , but the primary structure varies between species [36] , [37] . Thus, investigating how RNase T2 and h41 coevolve while maintaining their specific interaction should prove to be intriguing. In eukaryotes, the secondary structure of h41 is variable [36] , and whether the RNase T2-h41 interaction is possible remains unknown. Notably, in the gametophytic self-incompatibility system of Solanaceae, Rosaceae and Plantaginaceae, a male component, 'F-box protein', cancels the cytotoxic activity of non-self RNase T2 (the female component) [10] . Thus, in eukaryotes, the role of h41 as an RNase T2-inhibitor has probably been replaced by more sophisticated proteins during the course of evolution. In summary, we demonstrated that h41 of 16S rRNA recognizes RNase I through a specific interaction, which is the mechanism of RNase inhibition. This finding sheds light on the non-translational role of the 16S rRNA molecule. Because both RNase I (T2) and 16S rRNA are ubiquitous molecules, the origin of their interaction is surely ancient. Determining how these molecules have coevolved and promoted bacterial speciation will be of great interest. Plasmid construction Genomic DNA of Serratia ficaria (NBRC 102596) and Ralstonia pickettii (NBRC 102503) were extracted using the FastDNA Kit (BIO101). PCR amplification of their 16S rRNA genes (16S/Sfi or 16S/Rpi) was performed by KOD-Plus-Ver.2 DNA polymerase (Toyobo) using a pair of primers, Bac8f–UN1541r. This pair amplifies bacterial 16S rRNA genes from A8 to T1541 ( E. coli numbering), covering 99.5% of the gene [38] . pRB103/Eco carries an E. coli rrnB operon, Zeo r , and a pSC101 origin of replication [22] . To replace the 16S rRNA gene of Eco (16S/Eco) with 16S/Sfi or 16S/Rpi, we reverse-PCR-amplified the vector using the primer pair Bac8r–UN1541f. The product (7.9 kb) was ligated with 16S/Sfi or 16S/Rpi fragments using an In-Fusion Advantage PCR cloning Kit (Clontech), generating pRB103, in which the E. coli 16S rRNA gene was replaced with pRB103/Sfi or pRB103/Rpi. To replace the 3′-major domain of the 16S rRNA gene with its counterparts from Sfi or Rpi, we also made pRB103 constructs using the In-Fusion cloning strategy (for PCR primers, see Supplementary Table S1 ). For helix-swapping and mutational studies, we introduced mutations in 16S rRNA on pRB103 according to the Quik Change mutagenesis protocol [22] (for PCR primers, see Supplementary Table S1 ). E. coli genetic system KT101 (Δ rrnG Δ rrnA Δ rrnD Δ rrnE Δ rrnH Δ rrnB Δ rrnC /ptRNA67, pRB101), a derivative of SQ171 (Δ7 prrn strain) was used as a null mutant of the rrn operons of E. coli [22] , [23] . KT101 rna − is a derivative of KT101, in which rna (gene for RNase I) was inactivated by P1 transduction [22] . KT101 was maintained in 2× YT (1.6% (w/v) peptone, 1% (w/v) yeast extract and 0.5% (w/v) NaCl) medium supplemented with 50 μg ml −1 ampicillin (Amp) at 37 °C. Plasmid replacement strategy was performed as described elsewhere [22] . In short, KT101 or KT101 rna − was transformed with pRB103 constructs, followed by selection on LB plates supplemented with 100 μg ml −1 Zeocin (Zeo). To counter-select cells that had lost pRB101 (containing E. coli rrnB , sacB , Amp r , pSC101 ori), colonies were suspended in LB broth (100 μl), mixed well and spotted onto LB plates containing 100 μg ml −1 Zeo and 5% (w/v) sucrose. Through this procedure, only cells that contained a non- E. coli 16S rRNA gene could grow. We referred to the sucrose-resistant cells obtained thereby as KT103 (or KT103 rna − ) [22] . KT103 cells were grown at 37 °C in 2× YT medium supplemented with 100 μg ml −1 Zeo and 5% (w/v) sucrose. RNA extraction assay KT103 (or KT103 rna − ) cells (cultivated at 37 °C) were collected by centrifugation at 16,000 g for 2 min at 4 °C from 2 ml of culture when the turbidity reached OD 600 =0.5. Cells were washed once with ice-cold 10 mM Tris–HCl (pH 8.0) and resuspended in TE buffer (10 mM Tris–HCl, pH 8.0, 1 mM EDTA). The final turbidity was adjusted to OD 600 =5.0 and 100 μl of solution was used for RNA extraction analysis. In the EL method, lysozyme (chicken egg white; Sigma-Aldrich) was added to this solution to a final concentration of 40 μg ml −1 and incubated at 30 °C. After 6 min, the reaction was stopped by adding 1 ml of ISOGEN (phenol and guanidine thiocyanate-based reagent for RNA preparation [39] ; Nippon Gene), and RNA was extracted according to the manufacturer's instructions. During the 6-min incubation, periplasmic RNase I, which works even in the presence of EDTA, degrades RNA molecules, depending on the presence or absence of the inhibitory activity of the 30S subunit. In the direct extraction method, 1 ml of ISOGEN was added directly to Tris-washed cell pellets and cells were disrupted with glass beads by vigorous vortexing for 3 min. This procedure protects cellular RNA molecules from RNase I attack, regardless of the presence or absence of the inhibitory activity of the 30S ribosome. RNA electrophoresis RNA (OD 260 0.08, 3.2 μg; ∼ 8 μl) was mixed with 2 μl of 5× RNA loading buffer (80 mM MOPS, 4 mM EDTA, 2.7% (w/v) formaldehyde, 30.8% (w/v) formamide, 20 mM sodium acetate, 20% (v/v) glycerol, pH 7.0) and denatured for 5 min at 65 °C (ref. 22 ). Samples were electrophoresed on 1.2% formaldehyde–agarose gels [22] . Gels were stained with ethidium bromide. The digital image of each lane was analysed using the ImageJ 1.43u (Wayne Rasband) software and divided into ∼ 300 fractions ( x 1 – x ∼ 300 , where x 1 is at the bottom of the gel and x ∼ 300 the top): the signal intensity (RNA mass) of each fraction ( m 1 – m ∼ 300 ) was quantified. The centre of the RNA mass (as the degradation index) was calculated by the formula: x centre = m 1 x 1 + m 2 x 2 +... + m ∼ 300 x ∼ 300 /( m 1 + m 2 +...+ m ∼ 300 ). To compare x centre values between gels, the x -axis locations of bands corresponding to 23S rRNA and 5S rRNA/tRNAs were redefined as 100 and 0, respectively, and the recalculated x centre was marked by a green dot in each lane. In vitro inhibition assay To prepare ribosomal subunits, KT103 rna − derivatives were cultivated in 2 l of 2× YT medium supplemented with 100 μg ml −1 Zeo, 50 μg ml −1 Km and 5% (w/v) sucrose. Cells were disrupted by grinding with an equal amount of alumina powder [29] and suspended in RBS1 buffer (20 mM HEPES-KOH, pH 7.6, 30 mM NH 4 Cl, 4 mM Mg(OAc) 2 , 6 mM 2-mercaptethenol). Crude ribosome was prepared by two ultracentrifugation steps at 30,000 and 100,000 g (ref. 29 ). The 30S subunit was purified from crude preparations by sucrose density gradient centrifugation in RBS2 buffer (20 mM HEPES-KOH, pH 7.6, 500 mM NH 4 Cl, 0.5 mM Mg(OAc) 2 , 6 mM 2-mercaptethenol, 10–40% (w/v) sucrose) and resuspended in RBS1 buffer. Recombinant RNase I was purchased from New England Biolabs as a fusion with maltose-binding protein (molecular weight: 67 kDa). The inhibition assay was performed by mixing 0.4 OD 260 (28.8 pmol) of 30S subunit and 0.25 U of RNase I (0.075 pmol) in reaction buffer RB1 (100 μl; 50 mM Tris-HCl, pH 7.9, 100 mM NaCl, 10 mM MgCl 2 , 1 mM dithiothreitol). RNase I activity was measured at 30 °C using an RNase Alert Lab Test Kit (Ambion). Fluorescence (RFU: relative fluorescence units) was monitored using a SPECTRAmax GEMINI XS spectrofluorometer (Molecular Devices) with excitation/emission wavelengths of 490 nm and 520 nm, respectively. In vitro binding assay For the binding assay, 0.5 U of RNase I (0.15 pmol) was mixed with 0.4 OD 260 (28.8 pmol) of the 30S subunit in 120 μl of reaction buffer RB1. After 6 min of incubation at 30 °C, the reaction mixture was filtered through an Amicon Ultra 0.5-ml centrifugal filter (Millipore). Under these conditions, only free RNase I, and not the 30S subunit, was recovered from the flow-through fraction. Next, 100 μl of the flow-through fraction was used to detect RNase activity using the RNase Alert Lab Test Kit. Phenotype analysis An overnight (14 h) culture of KT103 (or KT103 rna − ) cells (100μ l) was inoculated into 100 ml of 2× YT medium supplemented with 100 μg ml −1 Zeo and 5% (w/v) sucrose and cultivated with rotation at 150 r.p.m. at 37 °C. To determine the growth curves of KT103 (or KT103 rna − ) cells on prolonged cultivation, a small amount of cultivation medium was removed at appropriate time points and the colony-forming units ml −1 on LB plates containing 100 μg ml −1 Zeo and 5% (w/v) sucrose were determined. Under our cultivation conditions (in the presence of 5% sucrose), KT103 (or KT103 rna − ) cells grew exponentially for the first 4 h, but usually continued to grow more slowly until 20 h (stationary phase). Total RNA was extracted by the direct extraction method using cells collected from 2 ml of cultivation medium sampled at 12 and 24 h. RNA samples were denatured and electrophoresed in a formaldehyde–agarose gel, followed by staining with ethidium bromide [22] . SrnB expression The gene encoding SrnB (118 bp) was synthesised and cloned into the expression vector pBAD [22] . This construct was used to transform KT103 (or KT103 rna − ) cells. Next, 100 μl of overnight (14 h) cultures of KT103 (or KT103 rna − ) cells transformed with the pBAD- srnB were inoculated into 100 ml 2× YT medium supplemented with 100 μg ml −1 Zeo, 50 μg ml −1 Amp and 5% (w/v) sucrose and cultivated in 500-ml Erlenmeyer flasks at 37 °C and 150 r.p.m. The turbidity of the culture was monitored in real-time (ODMonitor AS; Taitec). When the turbidity reached OD 600 =0.45, L -arabinose was added to a final concentration of 1 mM to induce SrnB expression. After 15 min, 2 ml of medium was sampled and total RNA was prepared by direct extraction. Samples were denatured and electrophoresed in a formaldehyde–agarose gel, followed by staining with ethidium bromide [22] . How to cite this article: Kitahara, K. & Miyazaki, K. Specific inhibition of bacterial RNase T2 by helix 41 of 16S ribosomal RNA. Nat. Commun. 2:549 doi: 10.1038/ncomms1553 (2011).